Lineage-restricted function of the pluripotency factor NANOG in stratified epithelia NANOG is a pluripotency transcription factor in embryonic stem cells; however, its role in adult tissues remains largely unexplored. Here we show that mouse NANOG is selectively expressed in stratified epithelia, most notably in the oesophagus where the Nanog promoter is hypomethylated. Interestingly, inducible ubiquitous overexpression of NANOG in mice causes hyperplasia selectively in the oesophagus, in association with increased cell proliferation. NANOG transcriptionally activates the mitotic programme, including Aurora A kinase ( Aurka ), in stratified epithelia, and endogenous NANOG directly binds to the Aurka promoter in primary keratinocytes. Interestingly, overexpression of Nanog or Aurka in mice increased proliferation and aneuploidy in the oesophageal basal epithelium. Finally, inactivation of NANOG in cell lines from oesophageal or head and neck squamous cell carcinomas (ESCCs or HNSCCs, respectively) results in lower levels of AURKA and decreased proliferation, and NANOG and AURKA expression are positively correlated in HNSCCs. Together, these results indicate that NANOG has a lineage-restricted mitogenic function in stratified epithelia. NANOG is a master transcription factor critical for the acquisition of both embryonic and induced pluripotency [1] . Nanog was discovered in embryonic stem cells (ESCs) for its ability to maintain ESCs self-renewal under conditions that would promote differentiation [2] , [3] , [4] . Accordingly, downregulation of Nanog in both mouse and human ESCs favours differentiation [1] , [5] , [6] . NANOG exerts its role in pluripotency in tight cooperation with two other pluripotency transcription factors, OCT4 (also known as POU5F1) and SOX2. Together, these three factors form a core transcriptional regulatory network essential for the acquisition and maintenance of ESC identity [7] , [8] , [9] , [10] , [11] , [12] . During mouse embryogenesis, these factors are highly expressed in the inner cell mass and their deletion causes early embryonic lethality [3] , [13] , [14] . Upon implantation, Nanog , Oct4 and Sox2 expression is silenced in the majority of tissues. OCT4 is not expressed in normal adult tissues, but it is a driving oncogene in germ cell tumours [15] , [16] . SOX2 is expressed in adult neural stem cells [17] and in specific epithelia, notably including the oesophagus and forestomach, where it plays a role in tissue homeostasis [18] . Interestingly, SOX2 is frequently overexpressed in human oesophageal and lung squamous carcinomas where it contributes a relevant oncogenic role [19] , [20] . Regarding NANOG, it is frequently overexpressed in a variety of human carcinomas [21] . However, there is a lack of systemic analyses on the role of NANOG in normal cells and adult tissues. In this study, first, we perform a comprehensive analysis of NANOG expression in adult mouse tissues and we observe that NANOG is selectively expressed in the basal layer of stratified epithelia, most prominently in the oesophagus. Second, we use an inducible transgenic mouse model to analyse the effects of NANOG overexpression in vivo , finding that NANOG induces hyperplasias in stratified epithelia, but not in other tissues, by activating pathways associated to mitosis. In particular, we identify the gene encoding the mitotic kinase AURKA as a relevant transcriptional target of NANOG in the oesophagus and in keratinocytes. Interestingly, overexpression of NANOG or AURKA in mice results not only in proliferation but also in aneuploidy. Finally, these findings are extended to human cancers derived from stratified epithelia. Altogether, we conclude that NANOG is a relevant regulator of cell proliferation whose activity is restricted to cells from stratified epithelia. NANOG is expressed in stratified epithelia We began by performing a systematic analysis of NANOG expression in adult mouse tissues. To simplify the interpretation of the data, we focused on the C57BL/6 strain because it does not carry any Nanog pseudogene with coding capacity [22] , [23] . Immunohistochemical staining of NANOG was negative in all major organs, including liver, lung, skeletal muscle, heart, intestine, kidney, testis and brain ( Fig. 1a , Supplementary Figs 1a and 3a ). In contrast, we observed clear NANOG-positive staining in the epithelium of the oesophagus, forestomach, mucosal tissues (oral, internal eyelid, vagina) and skin, and in the urothelium ( Fig. 1a,b , Supplementary Fig. 1a ). Positive staining was also observed in the myoepithelial layer of the mammary gland and prostate ( Supplementary Fig. 1a ). Similar results were obtained using two additional antibodies ( Supplementary Fig. 1b ). To further support the immunohistochemical data, we performed in situ hybridization (ISH) to detect Nanog RNA transcripts. In agreement with the immunohistochemistry (IHC) data, the epithelial layers of the oesophagus, forestomach and skin showed positive hybridization with the Nanog probe, whereas the underlying muscular and connective layers were negative ( Fig. 1a ). Nanog messenger RNA (mRNA) was undetectable in the liver ( Fig. 1a ). 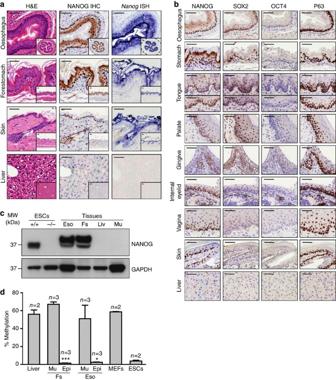Figure 1: NANOG expression in mouse adult tissues. (a) H&E staining, IHC for NANOG and ISH using aNanogRNA probe of the indicated adult tissues from C57BL/6 mice. Two magnifications are shown for each tissue. (b) IHC for NANOG, SOX2, OCT4 and P63 of the indicated adult tissues from C57BL/6 mice. Stomach corresponds to forestomach. Tongue shows the dorsal (upper) and ventral (lower) parts. (c) Immunoblot of NANOG extracts from the indicated tissues from C57BL/6 mice. Extracts from wild-type (+/+) andNanogknockout (−/−) ESCs are included as positive and negative controls and the amount loaded is one-tenth the amount loaded for the tissues. GAPDH was used as loading control. Eso, oesophagus; Fs, forestomach; Liv, liver; Mu, muscle, MW, molecular weight. (d) Methylation status of theNanogpromoter determined by pyrosequencing. Microdissected epithelial (Epi) and muscular (Mu) layers from forestomach (Fs) and oesophagus (Eso) from C57BL/6 mice (n=3 mice) were analysed. Liver was also analysed as a NANOG-negative tissue. MEFs (two independent isolates) and ESCs (two independent lines) were used as positive and negative controls, respectively. Values correspond to mean±s.e.m. Statistical significance was determined by the two-tailed Student’st-test comparing epithelial versus muscular layers: *P<0.05 and ***P<0.001. Inaandb, scale bars, 50 μm. Figure 1: NANOG expression in mouse adult tissues. ( a ) H&E staining, IHC for NANOG and ISH using a Nanog RNA probe of the indicated adult tissues from C57BL/6 mice. Two magnifications are shown for each tissue. ( b ) IHC for NANOG, SOX2, OCT4 and P63 of the indicated adult tissues from C57BL/6 mice. Stomach corresponds to forestomach. Tongue shows the dorsal (upper) and ventral (lower) parts. ( c ) Immunoblot of NANOG extracts from the indicated tissues from C57BL/6 mice. Extracts from wild-type (+/+) and Nanog knockout (−/−) ESCs are included as positive and negative controls and the amount loaded is one-tenth the amount loaded for the tissues. GAPDH was used as loading control. Eso, oesophagus; Fs, forestomach; Liv, liver; Mu, muscle, MW, molecular weight. ( d ) Methylation status of the Nanog promoter determined by pyrosequencing. Microdissected epithelial (Epi) and muscular (Mu) layers from forestomach (Fs) and oesophagus (Eso) from C57BL/6 mice ( n =3 mice) were analysed. Liver was also analysed as a NANOG-negative tissue. MEFs (two independent isolates) and ESCs (two independent lines) were used as positive and negative controls, respectively. Values correspond to mean±s.e.m. Statistical significance was determined by the two-tailed Student’s t- test comparing epithelial versus muscular layers: * P< 0.05 and *** P< 0.001. In a and b , scale bars, 50 μm. Full size image We compared the above-described pattern of NANOG expression with those of SOX2 and OCT4, which are the main transcriptional partners of NANOG in pluripotent cells [7] . Consistent with previous reports [16] , [18] , OCT4 was not detected in stratified epithelia, whereas SOX2 was clearly positive in the oesophagus, forestomach and oral mucosa, but weak in the internal eyelid, vagina and skin ( Fig. 1b ). As anticipated, the liver was negative for the three above transcription factors ( Fig. 1b ). Of note, NANOG and SOX2 are preferentially expressed in the basal layers of stratified epithelia and their expression patterns resemble those of the basal progenitor cell marker P63 ( Fig. 1b ). Also, we took advantage of the fact that teratomas contain undifferentiated areas together with a variety of differentiated structures, including stratified epithelia. As expected, teratoma undifferentiated areas were positive for NANOG, SOX2 and OCT4, and negative for the progenitor epithelial cell marker P63 ( Supplementary Fig. 1c ). On the other hand, teratoma areas of epithelial differentiation were positive for P63, and, interestingly, they were also positive for NANOG and SOX2, but negative for OCT4 ( Supplementary Fig. 1c ). Again, the staining for NANOG was reproduced using a total of three different antibodies ( Supplementary Fig. 1c ). To further validate our results, we performed immunoblots of total lysates from different tissues and we confirmed NANOG expression in the oesophagus and forestomach, but not in the liver or muscle ( Fig. 1c ). No other reactive bands were observed in the entire immunoblots ( Supplementary Fig. 2a ) and the same results were obtained with an additional antibody for NANOG ( Supplementary Fig. 2b ). As a control for the specificity of the anti-NANOG antibodies, we used wild-type (+/+) and Nanog -KO (−/−) ESC lysates [1] ( Fig. 1c , Supplementary Fig. 2a,b ). Of note, adult tissues presented two bands in the electrophoretic gels, which is in line with the complexity of NANOG transcriptional isoforms and post-transcriptional modifications [24] . To corroborate our data, we have generated Nanog -KO (−/−) chimeras using Nanog -KO (−/−) ESCs that carry a deletion of Nanog exons 2 and 3 and a green fluorescent protein (GFP) expression cassette under the control of the constitutively expressed CAG promoter [1] . Analysis of the chimeras showed that Nanog -KO (−/−) ESCs contributed to the coat hair ( Supplementary Fig. 2c ) and to the liver ( Supplementary Fig. 2d ). In contrast, Nanog -KO (−/−) ESCs did not contribute to the oesophagus and their contribution was residual in the epidermis ( Supplementary Fig. 2d ). The minimal contribution of Nanog -KO to stratified epithelia supports a functional role of NANOG in these tissues (see below). Finally, we wondered about the epigenetic status of the Nanog promoter in NANOG-positive epithelia. In particular, the differentially methylated region of Nanog is hypomethylated in pluripotent cells, such as ESCs, but it is heavily methylated in differentiated cells and in adult tissues, such as brain and testis, that do not express Nanog [25] , [26] , [27] , [28] . To investigate the DNA methylation status of the Nanog promoter in stratified epithelia, we microdissected the NANOG-positive basal layer of the oesophagus and forestomach, as well as the underlying NANOG-negative muscular layers. The extracted DNA was treated with bisulphite and directly subjected to pyrosequencing. We focused on two central CpG residues of the Nanog differentially methylated core region ( Supplementary Fig. 2e ). Importantly, similarly to ESCs, Nanog promoter was essentially devoid of methylation in the basal epithelial layers of the oesophagus and forestomach, whereas their respective adjoining muscular layers were methylated to the same extent as liver or mouse embryonic fibroblasts (MEFs) ( Fig. 1d ). In summary, multiple independent techniques (IHC, ISH, immunoblotting and DNA methylation) with positive and negative internal controls indicate that Nanog is expressed in the basal layer of stratified epithelia in adult mice. Nanog induces hyperplasia in stratified epithelia To interrogate the functional effects of NANOG in adult mice, we used a doxycycline (DOX)-inducible transgenic mouse model ( Col1a1::tetO-Nanog, ROSA26::rtTA ) ( Fig. 2a ), similar to a previously described Oct4 -inducible mouse model [29] . Upon increasing doses of DOX administration (0.2 mg ml −1 abbreviated ‘Lo’; and 2 mg ml −1 , ‘Hi’), we observed increasing levels of NANOG by ISH, IHC and immunoblotting in all tissues tested except the brain and testis that are poorly accessible to DOX ( Fig. 2b,c , Supplementary Fig. 3a ; see also below Fig. 3b , Supplementary Fig. 4a ). To assess the long-term impact of NANOG overexpression, we treated adult Col1a1 tetO-Nanog /+ ; ROSA26 rtTA /+ mice (abbreviated as ‘TG’) and their control littermates carrying only the transactivator Col1a1 +/+ ; ROSA26 rtTA /+ (abbreviated as ‘CTR’) with different doses of DOX and observed their phenotypic changes upon continuous administration. In the case of low DOX, half of the TG mice died within 16 weeks, and in the case of high DOX, the median survival was 6 weeks ( Fig. 2d ). Morbidity was accompanied by lower body weight ( Fig. 2e ), lower adiposity and lower bone mineral density ( Supplementary Fig. 3b,c ). 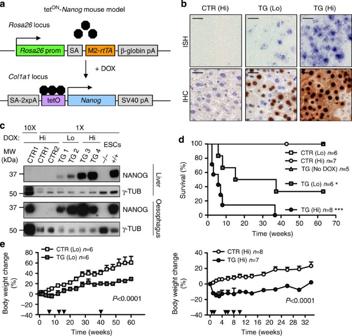Figure 2: InducibleNanogtransgenic mice. (a) Schematic representation of the knock-in alleles present inNanog-inducible mice. TheM2-rtTAgene was targeted into the ubiquitously expressedRosa26locus. A cassette containingNanogcDNA under the control of the DOX-responsive promoter (tetO) was inserted downstream of theCol1a1locus. SA, splice acceptor; pA, polyadenylation signal; tetO, tetracycline/DOX-responsive operator. Arrows indicate transcriptional start sites. (b) ISH using aNanogRNA probe and IHC for NANOG in liver sections (scale bars, 20 μm). CTR orNanog-overexpressing (TG) mice were analysed 72 h after administration of DOX in the drinking water at two different doses: 0.2 mg ml−1(Lo), and 2 mg ml−1(Hi). (c) Immunoblot of NANOG in the liver and oesophagus ofNanog-inducible mice treated with different doses of DOX. Samples from two independent mice were used for each condition, labelled CTR1, CTR2 and TG1 to TG4, as indicated. Two lanes were loaded with CTR1 extract: 1X, as all the other samples; and 10X, in the leftmost lane. Mice were treated with DOX, as inb, for 48 h. WT (+/+) andNanog-KO (−/−) ESCs were used as positive and negative controls. γ-TUB was used as a loading control. MW, molecular weight. (d) Survival curves ofNanog-inducible mice upon continuous treatment with DOX, as inb. TG mice not treated with DOX (No DOX) were also included as an additional control. Statistical significance was determined by the long-rank (Mantel-Cox) test (n, number of mice). TG (Lo) versus each of the three controls, *P<0.05. TG (Hi) versus each of the three controls, ***P<0.001. (e) Body weight change of CTR and TG mice continuously treated with DOX, as inb. All values are relative to the body weight at the start of the treatments (time 0). Arrow heads on the abscissae indicate killed animals that reached the humane endpoint. Values correspond to mean±s.e.m. of the indicated number of mice (n). Statistical significance was determined by two-way analysis of variance. Figure 2: Inducible Nanog transgenic mice. ( a ) Schematic representation of the knock-in alleles present in Nanog- inducible mice. The M2-rtTA gene was targeted into the ubiquitously expressed Rosa26 locus. A cassette containing Nanog cDNA under the control of the DOX-responsive promoter ( tetO ) was inserted downstream of the Col1a1 locus. SA, splice acceptor; pA, polyadenylation signal; tetO, tetracycline/DOX-responsive operator. Arrows indicate transcriptional start sites. ( b ) ISH using a Nanog RNA probe and IHC for NANOG in liver sections (scale bars, 20 μm). CTR or Nanog -overexpressing (TG) mice were analysed 72 h after administration of DOX in the drinking water at two different doses: 0.2 mg ml −1 (Lo), and 2 mg ml −1 (Hi). ( c ) Immunoblot of NANOG in the liver and oesophagus of Nanog -inducible mice treated with different doses of DOX. Samples from two independent mice were used for each condition, labelled CTR1, CTR2 and TG1 to TG4, as indicated. Two lanes were loaded with CTR1 extract: 1X, as all the other samples; and 10X, in the leftmost lane. Mice were treated with DOX, as in b , for 48 h. WT (+/+) and Nanog- KO (−/−) ESCs were used as positive and negative controls. γ-TUB was used as a loading control. MW, molecular weight. ( d ) Survival curves of Nanog- inducible mice upon continuous treatment with DOX, as in b . TG mice not treated with DOX (No DOX) were also included as an additional control. Statistical significance was determined by the long-rank (Mantel-Cox) test ( n , number of mice). TG (Lo) versus each of the three controls, * P< 0.05. TG (Hi) versus each of the three controls, *** P< 0.001. ( e ) Body weight change of CTR and TG mice continuously treated with DOX, as in b . All values are relative to the body weight at the start of the treatments (time 0). Arrow heads on the abscissae indicate killed animals that reached the humane endpoint. Values correspond to mean±s.e.m. of the indicated number of mice ( n ). Statistical significance was determined by two-way analysis of variance. 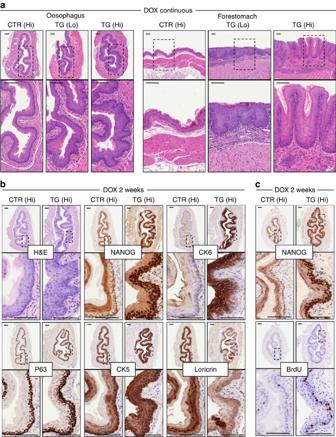Figure 3: NANOG overexpression causes hyperplasia in stratified epithelia. (a) H&E staining in the oesophagus (left) and forestomach (right) upon NANOG overexpression showing epithelial hyperplasia. CTR and TG mice were continuously treated with low or high DOX. Histological analyses were performed at the humane endpoint of TG mice (~2 months) or at the end of the observation period for CTR mice (11 months). (b) H&E and IHC of the indicated proteins in oesophageal serial sections of CTR and TG mice treated for 2 weeks with high DOX. (c) CTR and TG mice treated for 2 weeks with high DOX were injected intraperitoneally with BrdU 2 h prior to killing and oesophageal serial sections were analysed by IHC against NANOG and BrdU. In (a–c), pictures in the lower rows correspond to magnifications of selected areas in the upper pictures (marked with a dotted rectangle). Scale bars, 100 μm. Full size image Figure 3: NANOG overexpression causes hyperplasia in stratified epithelia. ( a ) H&E staining in the oesophagus (left) and forestomach (right) upon NANOG overexpression showing epithelial hyperplasia. CTR and TG mice were continuously treated with low or high DOX. Histological analyses were performed at the humane endpoint of TG mice (~2 months) or at the end of the observation period for CTR mice (11 months). ( b ) H&E and IHC of the indicated proteins in oesophageal serial sections of CTR and TG mice treated for 2 weeks with high DOX. ( c ) CTR and TG mice treated for 2 weeks with high DOX were injected intraperitoneally with BrdU 2 h prior to killing and oesophageal serial sections were analysed by IHC against NANOG and BrdU. In ( a – c ), pictures in the lower rows correspond to magnifications of selected areas in the upper pictures (marked with a dotted rectangle). Scale bars, 100 μm. Full size image To identify the pathological effects of NANOG overexpression, we performed an extensive histological analysis of TG and CTR mice at their time of death or at the experimental endpoint. The most striking alteration in TG mice was a marked hyperplasia of the oesophagus and forestomach ( Fig. 3a ). To better define the effects of NANOG overexpression before the onset of morbidity, we analysed TG and CTR mice that had been treated for 2 weeks with high DOX. We confirmed the induction of hyperplasia in the oesophagus and forestomach by NANOG overexpression, and mild hyperplasias were also observed in other stratified epithelia ( Fig. 3b , Supplementary Fig. 4a , Supplementary Table 1 ). In addition, the thymus was atrophic, which is consistent with the reported effect of Nanog overexpression in the hematopoietic system [30] . Alterations were also observed in the intestine (inflammation and Paneth cell mislocalization). The alterations in the oesophagus, stomach and intestine could impair nutrition and thus explain the reduced body weight. No significant changes were observed in major organs, such as liver, lung, heart, smooth and skeletal muscle, kidney, prostate and mammary gland ( Supplementary Fig. 4b , Supplementary Table 1 ). The lack of effect of NANOG on the functionality of liver and kidney was confirmed by normal blood levels of alanine transaminase (ALT) and total bilirubin (TBIL), respectively ( Supplementary Fig. 4c ). Nanog -induced hyperplasia in the oesophagus and forestomach was accompanied by expression of cytokeratin 6 ( Fig. 3b and Supplementary Fig. 4a ), which is characteristic of rapidly proliferating and hyperplastic squamous epithelial tissues [31] , [32] . We also observed an altered differentiation pattern, characterized by an expansion of basal layer markers P63 and CK5 into suprabasal layers, and by a reduced expression of the differentiation marker loricrin ( Fig. 3b ). Finally, we wondered if the hyperplastic phenotype was associated with the proliferation of basal epithelial cells. Indeed, BrdU-incorporation assays showed a striking increase in the number of proliferating basal cells of the oesophagus ( Fig. 3c , Supplementary Fig. 4d ). This was in contrast to the liver where NANOG overexpression did not impact on proliferation ( Supplementary Fig. 4b,d ). In summary, the most noticeable effects of NANOG are restricted to stratified epithelia, most prominently including the oesophagus, and, interestingly, these tissues correspond to those with high endogenous expression of NANOG. Mitotic activity of NANOG in stratified epithelia To understand the mechanisms underlying NANOG-induced hyperplasia in stratified epithelia, we treated TG mice and their control littermates with low or high DOX for only 48 h to capture early events triggered by NANOG. At this early time point, TG mice presented an increased proliferation in the basal and suprabasal layers of the oesophagus, measured by staining with Ki67 (which labels proliferative cells), by BrdU incorporation (which labels cells in S-phase) and by staining of phospho-histone 3 (pH3) (which labels cells in M phase) ( Fig. 4a,b ). A similar increase in Ki67-positive cells was also observed in the forestomach ( Supplementary Fig. 5a ). In the oesophagus, we also observed an increase in DNA damage, measured by phosphorylated H2AX (γH2AX), probably reflecting the induction of replicative stress by NANOG ( Fig. 4a ). Interestingly, we could not observe any increase in proliferation (Ki67, BrdU and pH3) or DNA damage in the liver, despite high overexpression of NANOG ( Supplementary Fig. 5b,c ). 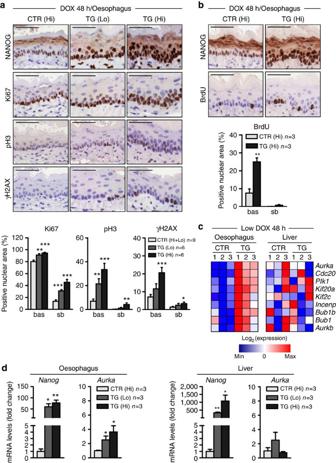Figure 4: Mitotic activity of NANOG in stratified epithelia. (a) IHC of NANOG, proliferation marker Ki67, mitotic marker pH3 and DNA damage marker γH2AX in oesophageal sections of CTR and TG mice treated with low or high DOX for 48 h. The graphs below correspond to the percentage of Ki67, pH3 and γH2AX-positive nuclear areas for each condition in the basal (bas) and suprabasal (sb) epithelial layers. CTR mice treated with low and high DOX were pooled (Hi+Lo). (b) IHC of NANOG and BrdU in oesophageal serial sections of CTR and TG mice treated, as ina, and injected intraperitoneally with BrdU 2 h prior to killing. The graph corresponds to the percentage of BrdU-positive nuclear areas for each condition in the basal (bas) and suprabasal (sb) epithelial layers. (c) Heat map of the expression of selected mitotic genes in the oesophagus and liver of CTR and TG mice treated with low DOX for 48 h. Values correspond to tissues from three independent mice, labelled 1–3. The colour intensity is proportional to the signal log2intensity: red upregulated and blue downregulated. (d) Relative gene expression in the oesophagus (left) and liver (right) ofNanogandAurkAdetermined by qRT–PCR. Mice (n=3) were treated as ina. Ina,b, scale bars correspond to 50 μm. Ina,b,d, values correspond to mean±s.e.m. of the indicated number of mice (n). Statistical significance was determined by the two-tailed Student’st-test: *P<0.05; **P<0.01; ***P<0.001. Figure 4: Mitotic activity of NANOG in stratified epithelia. ( a ) IHC of NANOG, proliferation marker Ki67, mitotic marker pH3 and DNA damage marker γH2AX in oesophageal sections of CTR and TG mice treated with low or high DOX for 48 h. The graphs below correspond to the percentage of Ki67, pH3 and γH2AX-positive nuclear areas for each condition in the basal (bas) and suprabasal (sb) epithelial layers. CTR mice treated with low and high DOX were pooled (Hi+Lo). ( b ) IHC of NANOG and BrdU in oesophageal serial sections of CTR and TG mice treated, as in a , and injected intraperitoneally with BrdU 2 h prior to killing. The graph corresponds to the percentage of BrdU-positive nuclear areas for each condition in the basal (bas) and suprabasal (sb) epithelial layers. ( c ) Heat map of the expression of selected mitotic genes in the oesophagus and liver of CTR and TG mice treated with low DOX for 48 h. Values correspond to tissues from three independent mice, labelled 1–3. The colour intensity is proportional to the signal log 2 intensity: red upregulated and blue downregulated. ( d ) Relative gene expression in the oesophagus (left) and liver (right) of Nanog and AurkA determined by qRT–PCR. Mice ( n =3) were treated as in a . In a , b , scale bars correspond to 50 μm. In a , b , d , values correspond to mean±s.e.m. of the indicated number of mice ( n ). Statistical significance was determined by the two-tailed Student’s t -test: * P< 0.05; ** P< 0.01; *** P< 0.001. Full size image Based on the above observations at such an early time point, we surmised that NANOG is directly implementing a proliferative transcriptional programme. To investigate this, we performed gene expression microarray analyses, at 48 h after low DOX, in total oesophagus and liver, which represent responsive and non-responsive tissues, respectively. Gene set enrichment analysis using public annotations from Reactome revealed that the overwhelming majority of pathways significantly upregulated by NANOG in the oesophagus were related to mitosis ( Supplementary Table 2 ), being the ‘M phase’ set the top upregulated pathway ( Supplementary Fig. 5d ). In contrast to the changes observed in the oesophagus, no pathways were significantly altered in liver. Inspection of the heat maps for individual genes present in the Reactome ‘M phase’ pathway suggested that NANOG could regulate the expression of pivotal mitotic genes specifically in the oesophagus but not in liver ( Fig. 4c ). Validation by quantitative PCR was obtained for Aurka , Aurkb , Kif20a and Bub1b , which showed upregulation upon NANOG induction in the oesophagus, but not in the liver ( Fig. 4d , Supplementary Fig. 5e,f ). These results indicate that NANOG enforces a proliferative programme selectively in the oesophagus. Aurka is a direct target of NANOG The above data on the transcriptional effects of NANOG in the oesophagus were based on the analysis of total oesophageal tissue, which includes epithelial and muscular layers. By IHC, we observed that NANOG induced an increase in AURKA-positive cells in the oesophageal epithelium, but not in the liver ( Fig. 5a ). 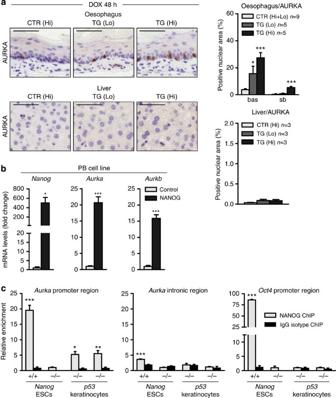Figure 5: NANOG binds and upregulates theAurkApromoter. (a) IHC of AURKA in oesophagus and liver sections of CTR and TG mice treated with high and low DOX for 48 h. Scale bars correspond to 50μm. The graphs to the right correspond to the percentage of AURKA-positive nuclear area for each condition in the basal (bas) and suprabasal (sb) epithelial layers of the oesophagus, or in the liver. CTR mice treated with low or high DOX were pooled (Hi+Lo). Values correspond to mean±s.e.m. of the indicated number of mice (n). Statistical significance was determined by the two-tailed Student’st-test: *P<0.05; ***P<0.001. (b) Relative mRNA levels of the indicated genes in PB cells transfected with a mouseNanogexpressing vector or mock transfected (control). Samples were analysed 72 h after transfection. Values correspond to mean±s.e.m. (n=3 technical replicates). Statistical significance was determined by the two-tailed Student’st-test: *P<0.05; ***P<0.001. (c) ChIP of NANOG in WT (+/+) orNanog-KO (−/−) ESCs or in primary WT (+/+) orp53-KO (−/−) keratinocytes. The relative recovery with respect to NANOG ChIP inNanog-KO ESCs is shown forAurkapromoter or intronic regions (seeSupplementary Fig. 6a), or for theOct4promoter region. In the case of keratinocytes, data from two independent biological replicates each from a different newborn mouse are shown. Values correspond to mean±s.e.m. of qPCR triplicates (Aurkapromoter or intronic regions) or duplicates (Oct4promoter). Statistical significance versus NANOG ChIP inNanog-KO (−/−) ESCs was determined by the two-tailed Student’st-test: *P<0.05; **P<0.01; ***P<0.001. Figure 5: NANOG binds and upregulates the AurkA promoter. ( a ) IHC of AURKA in oesophagus and liver sections of CTR and TG mice treated with high and low DOX for 48 h. Scale bars correspond to 50μm. The graphs to the right correspond to the percentage of AURKA-positive nuclear area for each condition in the basal (bas) and suprabasal (sb) epithelial layers of the oesophagus, or in the liver. CTR mice treated with low or high DOX were pooled (Hi+Lo). Values correspond to mean±s.e.m. of the indicated number of mice ( n ). Statistical significance was determined by the two-tailed Student’s t -test: * P< 0.05; *** P< 0.001. ( b ) Relative mRNA levels of the indicated genes in PB cells transfected with a mouse Nanog expressing vector or mock transfected (control). Samples were analysed 72 h after transfection. Values correspond to mean±s.e.m. ( n =3 technical replicates). Statistical significance was determined by the two-tailed Student’s t -test: * P< 0.05; *** P< 0.001. ( c ) ChIP of NANOG in WT (+/+) or Nanog -KO (−/−) ESCs or in primary WT (+/+) or p53 -KO (−/−) keratinocytes. The relative recovery with respect to NANOG ChIP in Nanog -KO ESCs is shown for Aurka promoter or intronic regions (see Supplementary Fig. 6a ), or for the Oct4 promoter region. In the case of keratinocytes, data from two independent biological replicates each from a different newborn mouse are shown. Values correspond to mean±s.e.m. of qPCR triplicates ( Aurka promoter or intronic regions) or duplicates ( Oct4 promoter). Statistical significance versus NANOG ChIP in Nanog -KO (−/−) ESCs was determined by the two-tailed Student’s t -test: * P< 0.05; ** P< 0.01; *** P< 0.001. Full size image To further explore the link between NANOG and aurora kinases, we recapitulated the above in vivo observations in a mouse keratinocyte cell line, PB [33] , [34] . Indeed, overexpression of NANOG resulted in a significant transcriptional upregulation of Aurka and Aurkb mRNA levels ( Fig. 5b ). Next, we wondered whether Aurka was a direct target of NANOG in epithelial cells. Inspection of the previously published chromatin immunoprecipitation (ChIP) data of NANOG in mouse ESCs [35] uncovered a NANOG binding site ~7 kb upstream of the Aurka transcriptional start site ( Supplementary Fig. 6a ). Based on this, we performed NANOG ChIP in WT (+/+) and Nanog -KO (−/−) ESCs and in primary mouse skin keratinocytes. For this, we took advantage of p53 -null (−/−) keratinocytes because of their robust proliferation and their higher basal levels of NANOG ( Supplementary Fig. 6b ), the latter being in agreement with the negative regulation of Nanog expression by p53 (ref. 36) [36] . We confirmed that NANOG binds the Aurka promoter in ESCs. Importantly, NANOG also bound the Aurka promoter in keratinocytes ( Fig. 5c ), whereas it did not bind to an intronic Aurka region or to the Oct4 promoter, which is not active in somatic tissues [16] . As a positive control, we confirmed that NANOG binds the Oct4 promoter in ESCs ( Fig. 5c ). We conclude that NANOG is acting as a direct transcriptional activator of the mitotic kinase AURKA and this function is conserved in ESCs and in stratified epithelia. Nanog and Aurka induce proliferation and aneuploidy AURKA is a kinase that has been extensively studied for its role in mitosis, although its functions go beyond mitosis, including the induction of DNA replication [37] . To evaluate the relevance of Aurka in mediating the effects of NANOG, we used an inducible transgenic mouse strain following the same strategy as the Nanog -inducible transgenic mice ( Col1a1::tetO-Aurka, ROSA26::rtTA ). We treated adult Col1a1 tetO-Aurka /+ ; ROSA26 rtTA /+ mice (abbreviated as ‘A-TG’) and their control littermates carrying only the transactivator Col1a1 +/+ ; ROSA26 rtTA /+ (abbreviated as ‘A-CTR’) with high doses of DOX for 48 h, and this resulted in an increase in AURKA-positive cells in the basal and suprabasal layers of the oesophagus ( Fig. 6a ) that was comparable to the level of AURKA-positive cells observed in Nanog transgenic mice (see Fig. 5a ). Interestingly, induction of Aurka elevated the proliferation rate of the basal cells of the oesophagus, measured by Ki67, BrdU incorporation and pH3 ( Fig. 6a ). After 2 weeks of induction, proliferation remained high in Aurka transgenic oesophagus, but this was not accompanied of a clear hyperplasia ( Fig. 6b ). Of note, the magnitude of the increase in BrdU incorporation and pH3 was lower upon Aurka overexpression compared with Nanog overexpression ( Figs 4a,b and 6a,b , Supplementary Fig. 4d ). Since the fraction of cells expressing AURKA is similar in Nanog and Aurka transgenice mice ( Figs 5a and 6a ), we conclude that AURKA contributes in part to the proliferative effects of NANOG together with a number of additional NANOG effectors, such as those revealed by our global analysis of mRNA levels ( Fig. 4c , Supplementary Table 2 ). 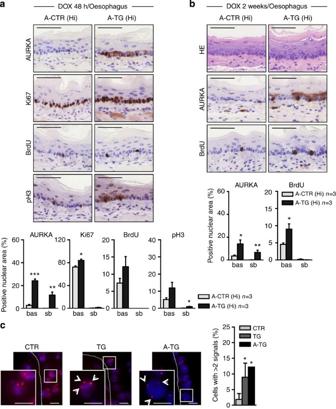Figure 6:NanogandAurkainduce proliferation and aneuploidy. (a) IHC of AURKA and the indicated proliferation markers in controlCol1a1+/+;Rosa26rtTA/+mice (A-CTR) andAurka-inducibleCol1a1tetO-Aurka/+;Rosa26rtTA/+(A-TG) littermate mice treated with high DOX for 48 h. The graphs below correspond to the percentage of AURKA, Ki67, BrdU and pH3-positive nuclear areas for each condition in the basal (bas) and suprabasal (sb) epithelial layers. (b) H&E staining, and IHC for AURKA and BrdU in oesophageal serial sections of A-CTR and A-TG mice treated for 2 weeks with high DOX and injected intraperitoneally with BrdU 2 h before killing. The graph shows the percentage of AURKA- and BrdU-positive nuclear areas for each condition in the basal (bas) and suprabasal (sb) epithelial layers. (c) Representative images of the oesophagus basal cells of CTR,Nanog-overexpressing (TG) andAurkA-overexpressing (A-TG) mice treated 2 weeks with high DOX, and hybridized against a chromosome 11 specific probe (white arrows). Dotted white lines mark the epithelial basal layer. Graph shows the quantification of cells showing more than two signals for the chromosome 11 probe. A total of 49 to 64 cells was quantified per group from a total of three CTR and TG mice, or one A-TG mouse. Statistical significance for the presence of more than two FISH signals (>2 signals) was determined using a two-sidedχ2test: *P<0.05. Inaandb, scale bars correspond to 50 μm; inc, scale bars correspond to 10 μm. Inaandb, values correspond to mean±s.e.m. of the indicated number of mice (n), and statistical significance relative to CTR was determined by the two-tailed Student’st-test: *P<0.05; **P<0.01; ***P<0.001. Figure 6: Nanog and Aurka induce proliferation and aneuploidy. ( a ) IHC of AURKA and the indicated proliferation markers in control Col1a1 +/+ ; Rosa26 rtTA/+ mice (A-CTR) and Aurka -inducible Col1a1 tetO-Aurka /+ ; Rosa26 rtTA/+ (A-TG) littermate mice treated with high DOX for 48 h. The graphs below correspond to the percentage of AURKA, Ki67, BrdU and pH3-positive nuclear areas for each condition in the basal (bas) and suprabasal (sb) epithelial layers. ( b ) H&E staining, and IHC for AURKA and BrdU in oesophageal serial sections of A-CTR and A-TG mice treated for 2 weeks with high DOX and injected intraperitoneally with BrdU 2 h before killing. The graph shows the percentage of AURKA- and BrdU-positive nuclear areas for each condition in the basal (bas) and suprabasal (sb) epithelial layers. ( c ) Representative images of the oesophagus basal cells of CTR, Nanog -overexpressing (TG) and AurkA -overexpressing (A-TG) mice treated 2 weeks with high DOX, and hybridized against a chromosome 11 specific probe (white arrows). Dotted white lines mark the epithelial basal layer. Graph shows the quantification of cells showing more than two signals for the chromosome 11 probe. A total of 49 to 64 cells was quantified per group from a total of three CTR and TG mice, or one A-TG mouse. Statistical significance for the presence of more than two FISH signals (>2 signals) was determined using a two-sided χ 2 test: * P< 0.05. In a and b , scale bars correspond to 50 μm; in c , scale bars correspond to 10 μm. In a and b , values correspond to mean±s.e.m. of the indicated number of mice ( n ), and statistical significance relative to CTR was determined by the two-tailed Student’s t -test: * P< 0.05; ** P< 0.01; *** P< 0.001. Full size image The overexpression of AURKA has been shown to produce aberrant mitosis and the consequent acquisition of chromosomal aneuploidies, and this could be a relevant driver for tumorigenesis [9] , [38] , [39] , [40] . Based on our above data, we hypothesized that Nanog overexpression, through the induction of Aurka and other mitotic inducers, should also result in aberrant mitosis and in the accumulation of aneuploid cells. Interestingly, Nanog or Aurka overexpression for 2 weeks resulted in abnormal mitotic figures in the oesophageal epithelium, which were absent in control samples ( Supplementary Fig. 6c ). Moreover, Nanog overexpression increased the number of aneuploid cells (>2 FISH signals for a chromosome 11 probe) to a similar extent as Aurka overexpression ( Fig. 6c ). These observations suggest that NANOG could contribute to tumorigenesis through the induction of aneuploidy caused by Aurka upregulation. NANOG is overexpressed in squamous cell carcinomas The mitogenic activity of NANOG in stratified epithelia prompted us to investigate the possible role of NANOG in squamous cell carcinomas. We began by exploring NANOG expression in archived mouse tumours. Interestingly, those tumours derived from stratified epithelia, such as forestomach, skin and vagina, were strongly positive for NANOG ( Fig. 7a ). Mammary and prostate tumours contained NANOG-positive cells, albeit of moderate intensity and restricted to a fraction of tumour cells ( Fig. 7a ). Tumours derived from NANOG-negative tissues, such as fibrosarcomas, intestinal adenomas and hepatocellular carcinomas, were completely negative for NANOG ( Fig. 7a ). These observations suggest that NANOG is strongly and widely expressed in cancers derived from stratified epithelia. 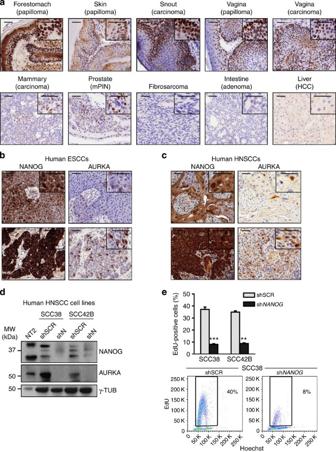Figure 7: NANOG is overexpressed in mouse and human squamous cancers. (a) NANOG IHC in archived mouse tumours. mPIN, mouse prostate intraepithelial neoplasia; (b) IHC of NANOG and AURKA in two representative human ESCCs. (c) IHC of NANOG and AURKA in two representative HNSCCs. (d) Immunoblots of HNSCC cells (SCC38 and SCC42B) infected with lentiviruses carrying scramble (shSCR) or anti-NANOG (shN) shRNAs. Samples were analysed 5 days after infection and selection. NTERA2 (NT2) cells were used as a positive control for NANOG. γ-tubulin (γ-TUB) was used as a loading control. MW, molecular weight. (e) Cells as indwere subjected to 1 h EdU pulse, Hoechst stained and analysed by flow cytometry. Their proliferation rate was quantified as the percentage of EdU-positive cells, see graph in the upper part of the panel. Values correspond to mean±s.e.m. of three (for SCC38) or two (for SCC42B) independent biological replicates. Statistical significance was determined by the two-tailed Student’st-test: **P<0.05; ***P<0.001. A representative flow cytometry plot is shown in the lower part of the panel. In (a–c), two magnifications are shown for each tissue and scale bars correspond to 50 μm. Figure 7: NANOG is overexpressed in mouse and human squamous cancers. ( a ) NANOG IHC in archived mouse tumours. mPIN, mouse prostate intraepithelial neoplasia; ( b ) IHC of NANOG and AURKA in two representative human ESCCs. ( c ) IHC of NANOG and AURKA in two representative HNSCCs. ( d ) Immunoblots of HNSCC cells (SCC38 and SCC42B) infected with lentiviruses carrying scramble (shSCR) or anti-NANOG (sh N) shRNAs . Samples were analysed 5 days after infection and selection. NTERA2 (NT2) cells were used as a positive control for NANOG. γ-tubulin (γ-TUB) was used as a loading control. MW, molecular weight. ( e ) Cells as in d were subjected to 1 h EdU pulse, Hoechst stained and analysed by flow cytometry. Their proliferation rate was quantified as the percentage of EdU-positive cells, see graph in the upper part of the panel. Values correspond to mean±s.e.m. of three (for SCC38) or two (for SCC42B) independent biological replicates. Statistical significance was determined by the two-tailed Student’s t -test: ** P< 0.05; *** P< 0.001. A representative flow cytometry plot is shown in the lower part of the panel. In ( a – c ), two magnifications are shown for each tissue and scale bars correspond to 50 μm. Full size image Based on the above, we decided to examine NANOG in human cancers derived from stratified epithelia. In humans, in addition to the NANOG1 gene characteristically expressed in ESCs, there is an almost identical paralog named NANOGP8 , which is fully functional in promoting pluripotency and it is often expressed in human cancer [41] . Given their almost identical protein sequence, currently available antibodies cannot distinguish between NANOG1 and NANOGP8 (the two proteins differ in two amino acids) and we refer to them collectively as NANOG. We focused on oesophageal squamous cell carcinomas (ESCCs) and head and neck squamous cell carcinomas (HNSCCs) for which there is evidence of NANOG expression [42] , [43] , [44] . We confirmed that NANOG expression is common in ESCCs ( n =29) and HNSCCs ( n =355), often with very intense and widespread staining, both in poorly differentiated and in well-differentiated carcinomas ( Fig. 7b,c , Supplementary Fig. 7a ). Of note, NANOG was also strongly positive in oesophageal samples with high-grade dysplasia and it was weakly positive in normal oesophagus ( Supplementary Fig. 7a ). The same series of cancers were stained for AURKA, which has been also found upregulated in ESCCs and HNSCCs [45] , [46] , [47] , [48] . We confirmed the presence of abundant AURKA-positive cells in both types of cancers ( Fig. 7b,c ). Interestingly, semiquantitative scoring of NANOG and AURKA indicated a positive association between these two proteins in HNSCCs (Spearman’s test ρ =0.386 and P <0.001; n =355). The AURKA gene is located in chromosome arm 20q, which is often amplified in many human cancers and contains multiple oncogenes [49] . We examined AURKA amplification in HNSCCs, but this was not associated with the intensity of AURKA staining ( Supplementary Fig. 7b ). Moreover, NANOG was also positively associated with Ki67 in HNSCCs (Spearman’s test ρ =0.560 and P <0.001; n =114). To establish a link between NANOG and AURKA mRNA levels, we silenced NANOG with a retroviral short hairpin RNA (shRNA) (sh NANOG ) in two human HNSCC cell lines that express NANOG to levels similar or higher than those in NTERA2 teratocarcinoma cells ( Supplementary Fig. 7c ). Importantly, knockdown of NANOG resulted in a concomitant decrease in AURKA in both cell lines ( Fig. 7d ), and this was accompanied by a decreased fraction of proliferating cells ( Fig. 7e ). Similar results on the levels of AURKA mRNA were observed in a NANOG-positive ESCC cell line upon silencing of NANOG ( Supplementary Fig. 7c,d ). These results indicate that AURKA expression is dependent on NANOG in human squamous carcinoma cells. Early studies based on total Nanog mRNA levels in whole-tissue extracts concluded that its expression was restricted to embryonic pluripotent cells [2] , [3] . In our current work, we have revisited this by specific staining of Nanog mRNA and protein in tissue sections. We have observed, using different antibodies, that NANOG is expressed in adult stratified epithelia, particularly, in the oesophagus, forestomach, skin, urothelium and mucosal tissues (oral and vagina). Moreover, we found that Nanog promoter is hypomethylated in the basal layer of the epithelium of the oesophagus and forestomach. Importantly, Nanog -null (−/−) ESCs did not contribute to the epithelia of the oesophagus in chimeric mice, whereas they contributed efficiently to the liver. Together these results indicate that NANOG could be functional in stratified epithelia. These findings are conceptually similar to those recently reported for the pluripotency factor SOX2, which also plays a relevant role in stratified epithelia [18] . Interestingly ubiquitous systemic expression of NANOG produced alterations that were restricted to those tissues with basal endogenous expression of NANOG. Most prominently, ectopic expression of NANOG caused a marked hyperplasia of the oesophagus and forestomach, characterized by an expansion of the basal layer. In contrast, other unrelated tissues, such as liver, with equal or superior levels of ectopic NANOG remained unaltered. Increased skin thickness has been recently reported upon overexpression of NANOGP8 in mice [50] . It is interesting to note that the basal layer of stratified epithelia contains the progenitor cells responsible for homeostatic tissue maintenance and this is particularly relevant in the case of the oesophagus, where progenitor cells constitute the only cell type responsible for the long-term maintenance of the tissue [51] , [52] . The lineage-restricted effect of NANOG is compatible with the existence of tissue-specific partners. Although the nature of these hypothetical partners is presently unknown, SOX2 is a good candidate due to its expression pattern [18] and its ability to interact with NANOG in ESCs [11] . The induction of oesophageal hyperplasia by NANOG suggests that it could promote proliferation in this tissue. Indeed, we observed that NANOG increased the proliferative activity of the oesophageal basal cells in a dose-dependent manner and soon after NANOG induction (48 h). Microarray analyses revealed that NANOG selectively induces a mitotic transcriptional programme in the oesophagus, but not in the liver. We focused in the critical mitotic inducer Aurora A kinase (AURKA), and we found that NANOG increases AURKA levels in the epithelial layer of the oesophagus, but not in the liver. Furthermore, overexpression or knockdown of NANOG in epithelial cell lines resulted in transcriptional upregulation or downregulation, respectively, of AURKA . Also, we found that NANOG directly binds the Aurka promoter in ESCs and in primary keratinocytes. To evaluate the potential of AURKA as an effector of NANOG, we examined Aurka -inducible mice. Interestingly, Aurka overexpression was able to induce proliferation of the basal layer of the oesophagus, although the effect was less pronounced than in the case of Nanog overexpression. These results suggest that Aurka is an important mediator of NANOG, but not the only one. Of note, high levels of AURKA have been associated to aberrant mitosis and to the ensuing acquisition of aneuploidy [9] , [38] , [39] , [40] . In support of the link between NANOG and AURKA, overexpression of Nanog or Aurka produced aberrant mitosis and aneuploidy in the oesophagus. These observations further reinforce the concept that Aurka is a relevant target of NANOG. Accumulating evidence indicates that embryonic pluripotency factors, such as OCT4 and SOX2, are highly expressed in particular human cancers [53] . Moreover, in the case of SOX2, which is expressed in adult stratified epithelia [18] , there is compelling evidence for its oncogenic role in human oesophageal squamous cell carcinomas (ESCCs) and mouse forestomach squamous cell carcinomas [19] , [54] . NANOG is also overexpressed in a number of human cancers, including ESCCs and head and neck squamous cells carcinomas (HNSCCs) [21] , [42] , [43] , [44] , [53] . Importantly, we have found a positive association between NANOG and AURKA expression in HNSCCs, suggesting that AURKA is a target of NANOG both in normal stratified epithelia and in their derived cancers. The expression of high levels of NANOG and AURKA in cancer could play an active role in neoplastic growth by increasing proliferation and chromosomal aberrations. In support of this, knockdown of NANOG in HNSCC cell lines decreased AURKA levels and the fraction of proliferating cells. In summary, our current study identifies a somatic function of NANOG in activating proliferation in stratified epithelia, and this function is retained in squamous cell carcinomas derived from stratified epithelia. Mice Mice were housed at the specific pathogen-free barrier area of the Spanish National Cancer Research Centre (CNIO), Madrid. Mice were observed on a daily basis and killed when they showed overt signs of morbidity in accordance to the Guidelines for Humane Endpoints for Animals Used in Biomedical Research from the Council for International Organizations of Medical Sciences (CIOMS). All animal procedures were performed according to protocols approved by the CNIO-ISCIII Ethics Committee for Research and Animal Welfare (CEIyBA). The attention-inducible mice, generated and kindly provided by Konrad Hochedlinger and Rudolf Jaenisch, carried the M2-rtTA gene inserted within the Rosa26 allele and a cassette containing the Nanog cDNA under the control of the DOX-responsive promoter ( tetO ) inserted downstream of the Col1a1 locus, as described elsewhere for the generation of OCT4-inducible mice [29] . The Aurora kinase A ( AurkA )-inducible mice used in this work has been generated following the same strategy used for the generation of Nanog -inducible mice and their detailed characterization will be published elsewhere. The final mouse model Col1a1 tetO-Aurka/+ ;Rosa26 rtTA/+ , named A-TG, overexpresses exogenous AurkA upon DOX treatment in a wide range of proliferative and non-proliferative tissues. We used wild-type 100% pure C57BL/6 mice, 3–5 weeks of age and of both sexes indistinguishably in the following figures ( Fig. 1a–d , Supplementary Figs 1a and 2a,b ), and we used control Col1a1 +/+ ; Rosa26 rtTA/+ or Col1a1 tetO-Nanog /+ ; Rosa26 +/+ (CTR and A-CTR), Nanog -inducible Col1a1 tetO-Nanog /+ ; Rosa26 rtTA/+ (TG) and AurkA -inducible Col1a1 tetO-AurkA /+ ; Rosa26 rtTA/+ (A-TG) littermate mice of mixed 129Sv;C57BL/6 background, 3–8 months of age and of both sexes indistinguishably, for the following figures ( Figs 2 , 3 , 4 , 5 , 6 , Supplementary Figs 3–6 ). Transgene expression was induced in mice by replacing normal drinking water with 7.5% sucrose solution containing DOX (0.2 mg ml −1 (low DOX) or 2 mg ml −1 (high DOX)). For prolonged treatment, mice were treated with low DOX and 2% sucrose or with high DOX and 7.5% sucrose and the DOX-containing water was changed every 2–3 days. Generation of chimeric mice For chimera generation, 5–6 Nanog -KO (−/−) ESCs (RCNßH(t); GFP-positive; agouti coat; kindly provided by Ian Chambers) [1] were microinjected into C57BL/6J ( Nanog WT, GFP negative, black coat) or into C57BL/6- Tyr c-2J /J ( Nanog WT, GFP negative, white coat) E3.5 blastocysts. Chimerism was determined by coat colour. In vivo BrdU incorporation assay Bromodeoxyuridine (5-bromo-2′-deoxyuridine) was purchased from Sigma (B9285) and was diluted to 100 mg ml −1 in physiological serum (0.9% w/v NaCl). We treated TG mice (both TG and A-TG) and their control littermates with high DOX for 48 h or 2 weeks and, 2 h before killing, mice received a single intraperitoneal injection of BrdU at 100 μg g −1 of body weight. Cell culture Wild-type ESCs and Nanog -KO (−/−) ESCs (see above ‘Generation of chimeric mice’) were grown under 3% O2 tension in DMEM (high glucose) supplemented with 15% KnockOut Serum Replacement (Invitrogen), leukaemia inhibitory factor 1,000 μ ml −1 , 2i (CHIR99021 (1 μM) and PD0325901 (1 μM), Axon Medchem), non-essential amino acids, glutamax and ß-mercaptoethanol. ESCs were routinely grown on feeder cells. For analyses, ESCs were adapted to gelatin-coated plates for at least three passages, and this was done in the absence of 2i. Primary mouse embryonic fibroblasts were obtained from E13.5 C57BL/6 embryos. Mouse embryonic fibroblasts, murine-transformed keratinocyte cell line PB [33] , [34] (a kind gift of Jesus Paramio), human NTERA2 teratocarcinoma cells, oesophageal cancer cell lines TE1 and TE2 (ref. 55) [55] (a kind gift of Anil Rustgi), and human HNSCC cell lines Cal27, Cal33 and HN6 (refs 56 , 57 ) (a kind gift of J. Paramio) and SCC40, SCC38, SCC29, SCC42B and SCC2 (ref. 58) [58] (a kind gift of Reidar Grénman), were all grown in (DMEM) (Gibco) supplemented with 10% fetal bovine serum (Hyclone) and antibiotic–antimycotic solution (Gibco). Primary keratinocytes were freshly isolated from p53 -null (−/−) [59] C57BL/6 neonates (days 1–4 postpartum). After dispase (STEMCELL Technologies) treatment, the epidermis was separated from the dermis, minced and stirred. The derived cell suspension was then filtered through a sterile teflon mesh (Cell Strainer 0.7 μm, Falcon) to remove cornified sheets and keratinocytes were collected by centrifugation (160 g ) and seeded on collagen I precoated cell culture plates (BD Biosciences). Keratinocytes were cultured in Cnt-07 (CELLnTEC) medium supplemented with antibiotic–antimycotic solution (Gibco). Cultures were routinely tested for mycoplasma and were always negative. RNA in situ hybridization For RNA ISH [60] , mouse tissues were fixed overnight in 4% paraformaldehyde, embedded in paraffin and cut in 7-μm thick sections. After rehydration and refixing, sections were permeabilized with Proteinase K followed by mild HCl treatment and washed with phosphate-buffered saline (PBS). Sections were prehybridized for 2 h at 65 °C, and then hybridized overnight at 65 °C in the dark. ISH was carried out using a mouse Nanog anti-sense probe. This probe corresponds to the complete coding region of the mouse Nanog gene (positions 216–1133 of RefSeq NM_028016) cloned as a PCR product in the pCRII-TOPO cloning vector (Invitrogen). The vector was linearized with Bam HI and transcribed using T7 RNA polymerase in the presence of DIG labelled nucleotides. Sections were extensively washed and incubated with an anti-DIG alkaline phosphates linked Fab fragments (Roche) overnight at 4 °C. After further washes, colour reaction was developed with the chromogenic BM-purple substrate (Roche). Sections were washed, spot-fixed with 4% paraformaldehyde and mounted. Digital slides were acquired with a MIRAX SCAN (Zeiss) and images were captured with the Pannoramic Viewer Software (3DHISTECH). Analysis of aneuploidy by fluorescence ISH (FISH) OCT oesophageal cryosections (5 μm thick) were adhered to glass slides and digested in 0.5% pepsin in 0.2 N HCl for 10 min at 37 °C. Slides were incubated in methanol:acetic acid (3:1) for 10 min at room temperature (RT) and then dehydrated for 4 min each in 70, 85 and 100% ethanol. Two pericentromeric probes from mouse chromosome 11 (RP23-478B14 and RP23-263C13) were labelled with Red-dUTP using nick translation. Probes were denatured by incubation for 5 min at 90 °C and then applied to dried slides, which were covered with coverslips and incubated at 75 °C for 3 min. Sealed slides were incubated overnight at 37 °C in a humidified chamber and then washed for 2 min at 75 °C in 0.8 × SSC, 0.3% NP-40 and for 5 min at RT in 2 × SSC. Cells were stained with 4′,6-diamidino-2-phenylindole washed with PBS and mounted using Prolong. Image stacks were acquired on a Leica D3000 fluorescence microscope and flattened into a maximal projection before being scored. Chromosome gains (>2 FISH signals) were counted. Histopathology and IHC in mice Tissue samples were fixed in 10% buffered formalin, embedded in paraffin and sectioned at a thickness of 2.5 μm. Consecutive sections were stained with hematoxylin and eosin (H&E) and processed for IHC performing antigen retrieval in a VENTANA DISCOVERY XT (Roche) with CC1 buffer and incubating them with the following three antibodies against NANOG: Novus Biologicals, NB100-58842 lot #5-1, 1/50 (stock 1 mg ml −1 ); Calbiochem, SC1000, 1/150 (stock 1 mg ml −1 ); and CNIO-NF238 in-house made rat monoclonal antibody against full-length mouse NANOG, supernatant 1/2. When not specified, the anti-NANOG antibody used is the one from Novus Biologicals. Other antibodies used recognized: SOX2 (Cell Signaling, C70B1), 1/50; OCT4 (Abcam, Ab19857), 1/500 (stock 1 mg ml −1 ); P63 (Sigma, P3737), 1/750 (stock 0.2 mg ml −1 ); CK6 (Covance, PRB-169P), 1/1,000 (stock 1 mg ml −1 ); CK5 (Covance, PRB-160P), 1/5,000 (stock 1 mg ml −1 ); LORICRIN (Covance, PRB-145P), 1/500 (stock 1 mg ml −1 ); Ki67 (Master Diagnóstica, 000310QD), ‘ready to use’; γH2AX (Millipore, 05-636), 1/5,000 (stock 1 mg ml −1 ); AURKA (Becton Dickinson, San Jose, CA, 610938), 1/100 (stock 0.25 mg ml −1 ); pH3 (Ser10) (Millipore, 06-570), 1/500 (stock 1 mg ml −1 ); and bromodeoxyuridine (GE Healthcare, RPN202), 1/100. Following incubation with the primary antibodies, positive cells were visualized using 3,3′-diaminobenzidine tetrahydrochloride plus as a chromogen. Counterstaining was performed with hematoxylin. Digital slides were acquired with a MIRAX SCAN (Zeiss), images captured with the Pannoramic Viewer Software (3DHISTECH) and image analysed and quantified with the AxioVision software (Zeiss). Immunofluorescence For tissues, paraffin-embedded sections were deparaffinized and antigen retrieval was performed. Sections were blocked with 1% fetal bovine serum for 1 h at RT, and then incubated for 2 h at RT with NANOG antibody (Novus Biologicals, NB100-58842 lot #5-1, 1/50, stock 1 mg ml −1 ) in Dako Antibody Diluent with Background Reducing Components. After washing (three times with PBS 0.1% Triton X-100), the procedure was repeated using GFP antibody (Roche 11814460001, 1/50, stock 0.4 mg ml −1 ). Slides were then stained with donkey anti-rabbit AlexaFluor555-conjugated secondary antibody for NANOG and with goat anti-mouse AlexaFluor488-conjugated secondary antibody for GFP (both secondary antibodies from Invitrogen) in Dako REAL buffer, 1 h at RT, followed by 4′,6-diamidino-2-phenylindole staining to visualize the nuclei. Slides were mounted with Vectashield antifade medium (Vector Laboratories) before confocal analysis. Confocal microscopy was performed with a TCS SP5 laser scanning spectral microscope (Leica Microsystems) equipped with a Plan-Apochromat × 40/1.2 NA oil objective. Eight-bit images were acquired using the Leica LAS AF v.2.1 software (Leica Microsystems). The pictures show the maximum projection of Z -stacks. Bisulphite pyrosequencing The NANOG-positive layer of the oesophagus and forestomach, as well as, the underlying NANOG-negative layers were microdissected using serial sections stained with NANOG or with H&E. The NANOG-stained section was used to create a mask that was applied to the H&E section for microdissection using a PALM MicroBeam (Zeiss). Genomic DNA isolation from microdissected samples was performed with RecoverAll Total Nucleic Acid Isolation Kit (Ambion). Bisulphite modification of DNA was performed with the EZ DNA Methylation-Gold kit (Zymo Research) following the manufacturer’s instructions. Primers for PCR amplification and sequencing were designed to flank CpG sites −292 and −301 (relative to the start codon of Nanog ENSEMBL ENSMUST00000012540, see Supplementary Fig. 2e ) and to hybridize with CpG-free sites to ensure methylation-independent amplification, using the software PyroMark Assay Design (version 2.0.01.15; Qiagen, Hilden, Germany). Primer sequences are provided in the Supplementary Table 3 . PCR was performed with primers biotinylated to convert the PCR product to single-stranded DNA templates, using the Vacuum Prep Tool. Pyrosequencing reactions and methylation quantification were performed using PyroMark Q24 reagents, equipment and software (version 2.0.6; Qiagen), according to manufacturer’s instructions. Microarrays Total RNA was extracted from the oesophagus using RNeasy Fibrous Tissue Mini Kit (Qiagen), and from liver by combining an initial lysis with Trizol (Invitrogen) with a clean-up with RNeasy Kit (Qiagen). Total RNA was labelled with the One-Color Microarray-Based Gene Expression Analysis (Quick Amp Labeling) kit (Agilent). Samples were hybridized to Whole Mouse Genome 4x44K microarrays (Agilent) by following the manufacturer’s instructions. Microarrays were scanned on a G2565C DNA microarray scanner (Agilent) and images were analysed with Feature Extraction Software (version 10.1.1). Microarray background subtraction was carried out using normexp method. To normalize the data set, we performed loess within arrays normalization and quantiles between arrays normalization. Gene set enrichment analysis [61] was applied using annotations from Reactome. Genes were ranked based on limma moderated t statistic. After Kolmogorov–Smirnoff test, only those gene sets showing false discovery rate <0.05 were considered enriched between classes under comparison. Quantitative real-time PCR In the case of cultured cells, total RNA was obtained using RNeasy Mini Kit (Qiagen) following the manufacturer’s instructions. In the case of the oesophagus or liver, total RNA was isolated as stated above (see ‘Microarrays’). RNA samples were treated with DNase I (Qiagen) before reverse transcription. To generate cDNA, total RNA was reverse transcribed using random priming and Superscript Reverse Transcriptase (Life Technologies), according to the manufacturer’s protocols. Primer sequences are provided in Supplementary Table 3 . Quantitative real-time PCR was performed using DNA Master SYBR Green I mix (Applied Biosystems, Foster City, CA) in an ABI PRISM 7700 qthermocycler (Applied Biosystems). Calculation for the values was according to the ΔΔ C T method [62] and using Gapdh/GAPDH as control. Immunoblotting Nuclear protein extracts were prepared using the Nuclear/Cytosol Fractionation kit (BioVision) following protocols provided by the manufacturer. Total lysates were prepared using lysis buffer (50 mM Tris–HCl pH 7.5, 150 mM NaCl, 4 mM CaCl 2 , 1.5% Triton X-100, protease inhibitors and micrococcal nuclease). In the case of tissue extracts, lysates were homogenized using a Precellys 24 tissue homogenizer. For western blot analysis, protein extracts were resolved using NuPAGE 4–12% gradient Bis-Tris gels, transferred to nitrocellulose and incubated with the corresponding antibodies. For mouse NANOG detection, we used a total of three different antibodies: Novus Biologicals, NB100-58842 lot #5-1, 1/1,000 (stock 1 mg ml −1 ); Calbiochem, SC1000, 1/1,000 (stock 1 mg ml −1 ); and Millipore, AB9220, 1/2,000 (stock 1 mg ml −1 ). When not specified, the anti-NANOG antibody used for immunoblots is the one from Novus Biologicals. For human NANOG detection, we used Cell Signaling, D73G4, 1/1,000. Other antibodies used recognized: p53 (Leica, NCL-P53-CM5P), 1/200; histone H3 (Abcam, Ab1791), 1:2,000 (stock 1 mg ml −1 ); total AURKA (IAK1, BD Biosciences, 610938), 1/1,000 (stock 0.25 mg ml −1 ); γ-tubulin (Sigma, GTU-88), 1/10,000; GAPDH (Sigma, G8795), 1/2,000 (stock 1 mg ml −1 ); and SMC-1 (Bethyl, A300-055A), 1/10,000 (stock 1 mg ml −1 ). Uncropped scans of the blot images are presented in Supplementary Figs 2a and 8 . ChIP Cells were cross-linked with 1% formaldehyde for 15 min at RT. Cross-linking was stopped by the addition of glycine to a final concentration of 0.125 M. Fixed cells were lysed in lysis buffer (1% SDS, 10 mM EDTA, 50 mM Tris–HCl, pH 8.0 and protease inhibitors) and sonicated. As input, 60 μg of protein extract was reserved. For immunoprecipitation, 600 μg of protein was diluted to 1 ml with dilution buffer (1.1% Triton X-100, 0.01% SDS, 1.2 mM EDTA, 167 mM NaCl and 16.7 mM Tris–HCl, pH 8.0 and protease inhibitors), precleared with A/G plus-agarose preblocked with bovine serum albumin (Santa Cruz) and incubated with an antibody against mouse NANOG (Novus Biologicals, NB100-58842 lot #5-1, 1/250, stock 1 mg ml −1 ) or with rabbit IgG isotype (Jackson ImmunoResearch, 011-000-003, 1/2750, stock 11 mg ml −1 ). Immune complexes were precipitated with A/G plus-agarose pre-blocked with bovine serum albumin and washed sequentially with low-salt immune complex wash buffer (0.1% SDS, 1% Triton X-100, 2 mM EDTA, 150 mM NaCl, 20 mM Tris–HCl pH 8.0), high-salt immune complex wash buffer (0.1% SDS, 1% Triton X-100, 2 mM EDTA, 500 mM NaCl, 20 mM Tris–HCl, pH 8.0), LiCl immune complex wash buffer (0.25 M LiCl, 1% NP-40, 1% deoxycholate-Na, 1 mM EDTA, 10 mM Tris–HCl, pH 8.0) and TE buffer (1 mM EDTA, 10 mM Tris–HCl pH 8.0), and finally eluted in elution buffer (1% SDS, 50 mM NaHCO 3 ). All samples, including inputs, were subjected to reverse cross-linking, treated with proteinase K and DNase-free RNase and DNA was extracted with QIAGEN PCR purification column (Qiagen) and resuspended in TE buffer. Primer sequences are provided in Supplementary Table 3 . Metabolic analyses Blood was collected from the submandibular vein and blood levels of alanine transaminase (ALT) and total bilirubin were determined using VetScan rotors (Abaxis Veterinary Diagnostics). Cell transfection For NANOG silencing, TE2 human oesophageal cancer cells were transfected with a pool of four siRNA duplexes targeting NANOG ( ON-TARGETplus Human NANOG (79923) siRNA, SMARTpool, Dharmacon) or with a pool of scramble siRNA duplexes (ON-TARGET plus Non-targeting Control Pool, SMARTpool, Dharmacon) using Lipofectamine RNAiMAX in Opti-MEM I (Invitrogen) according to the manufacturer’s instructions. Cells were processed for RNA extraction 48 h after transfection. For NANOG overexpression, murine-transformed keratinocyte cell line PB was transfected with the mouse NANOG expressing plasmid pPyCAG-Nanog-IP (Addgene plasmid #13838) [3] using Fugene HD transfection reagent (Promega) according to the manufacturer’s protocol. Cells were processed for RNA extraction 72 h after transfection. Lentiviral transduction of shRNAs Lentiviruses containing pLKO.1-scramble shRNA (shSCR), and pLKO.1-NANOG-shRNA vectors (TRCN000004885, TRCN000004886 and TRCN000004887) obtained from Open Biosystems (Thermo Scientific Open Biosystems) were produced in 293T cells using the lentivirus packaging plasmids pLP1, pLP2 and pLP/VSVG (Invitrogen), by co-transfecting all plasmids using Fugene HD transfection reagent (Promega) according to the manufacturer’s protocol. Cells were plated the day prior to infection, and supernatants were collected 48 h from 293T cells after transfection. Cell lines SCC38 and SCC42B were infected concomitantly with all three lentiviruses that target NANOG to obtain a synergic silencing effect. Cells were selected with puromycin to obtain shSCR and sh NANOG cell lines. Cells were analysed 5 days after starting infections. EdU labelling Cells were pulsed for 1 h with 10 μM of EdU (5-ethynyl-2′-deoxyuridine) and then collected, fixed in 4% PFA and processed following the Click-iT protocol (Invitrogen). Samples were run in a BD FACSCanto II (Becton Dickinson) equipped with a 488 and 407 nm lines, and at least 10,000 single events were recorded. All data were analysed using FlowJo v9.7.5 (Treestar, Oregon). Analysis of human cancers Oesophageal and HNSCCs were collected and handled anonymously at collaborating institutions (University College London Hospital, Hospital Clinic of Barcelona, and Hospital Universitario Central de Asturias) with the approval of their institutional review boards and following standard ethical and legal protection guidelines regarding human subjects, including informed consent for all the subjects. Consecutive paraffin sections were processed for IHC in a Leica Bond III (Leica) or in Dako Autostainer Plus (Dako) with antibodies against human NANOG (Cell Signaling, D73G4, 1/50), AURKA (Novocastra, NCL-L-AK2, supernatant 1/100) or and Ki67 (Dako, clone MIB-1, ‘ready to use’). Following incubation with the primary antibodies, positive cells were visualized using 3,3′-diaminobenzidine tetrahydrochloride plus as a chromogen. Counterstaining was performed with hematoxylin. Digital slides were acquired with a MIRAX SCAN (Zeiss), images captured with the Pannoramic Viewer Software (3DHISTECH). Slides were scored by a trained pathologist. For NANOG staining, a semiquantitative scoring system based on staining intensity was applied: negative (0), weak (1) and strong protein expression (2). AURKA immunostaining was quantified as follows: quantity scores from 0 to 3 were respectively assigned if 0%, <10%, 10–50% or >50% of the tumour cells were positive; staining intensity was rated on a scale of 0–2 (0=negative, 1=weak and 2= strong). The raw data were then converted to a German Immunoreactive Score by multiplying the quantity and staining intensity scores. Immunostaining for Ki67 was evaluated using quantity scores from 0 to 4 assigned respectively if 0%, 1–25%, 26–50%, 51–75%, and 76–100% of nuclei were stained. Correlations between NANOG, AURKA and Ki67 were tested by two-sided Spearman’s correlation coefficient. Amplification analysis of the AURKA gene DNA was extracted from formaldehyde-fixed, paraffin-embedded tissues punches by applying an extraction protocol [63] , which includes thorough deparaffinization with xylene, methanol washings to remove all traces of the xylene and a 24-h incubation in 1 mol l −1 sodium thiocyanate to reduce cross-links. Subsequently, the tissue pellet was digested for 3 days in lysis buffer with high doses of proteinase K (final concentration, 2 μg μl −1 , freshly added twice daily). Finally, DNA extraction was done by using the QIAamp DNA Mini Kit (Qiagen). AURKA gene amplification was evaluated using quantitative real-time PCR in an ABI PRISM 7500 Sequence detector (Applied Biosystems) using Power SYBR Green PCR Master Mix. Primer sequences are provided in Supplementary Table 3 . Amplification-positive cases were confirmed using a second reference gene HNMT located at 2q22.1. Samples were analysed in triplicates and template-free blanks were also included. Dissociation curve analysis of all PCR products showed a single sharp peak and the correct size of each amplified product was confirmed by agarose gel electrophoresis. The relative gene copy number for AURKA was calculated using the 2 −ΔΔ C T method [62] . The ΔΔ C T represents the difference between Δ C T of tumour −Δ C T of normal epithelia, with Δ C T being the average C T for the target gene ( AURKA ) minus the average C T for the reference gene ( TH or HNMT ). Values higher than 2.0 were considered positive for gene amplification. Genomic DNA isolated from DLD1 and Caco-2 cell lines, respectively served as negative and positive control for AURKA gene amplification [64] . Statistical analysis Sample size for animal experimentation followed Mead’s recommendations in the large majority of assays [65] . Samples (cells or mice) were allocated to their experimental groups according to their predetermined type (cell type or mouse genotype) and therefore, there was no randomization. Investigators were not blinded to the experimental groups (cell types or mouse genotypes) and no mice were censored. Values were expressed as mean ± s.e.m. and differences with P value <0.05 were considered significant (* P <0.05, ** P <0.01, *** P <0.001). Comparisons between two groups were performed using unpaired two-tailed Student’s t- test. For the experiment in Fig. 6c , statistical significance was determined using a two-sided χ 2 test. For survival curves, we used the Long-rank (Mantel-Cox) test. Time courses were analysed by two-way analysis of variance. These statistical analyses were performed using GraphPad Prism software. Accession codes : The raw microarray data have been deposited in the Gene Expression Omnibus repository under accession number GSE48370 . How to cite this article : Piazzolla, D. et al. Lineage-restricted function of the pluripotency factor NANOG in stratified epithelia. Nat. Commun. 5:4226 doi: 10.1038/ncomms5226 (2014).